Construction of RNA nanocages by re-engineering the packaging RNA of Phi29 bacteriophage RNA nanotechnology promises rational design of RNA nanostructures with wide array of structural diversities and functionalities. Such nanostructures could be used in applications such as small interfering RNA delivery and organization of in vivo chemical reactions. Though having impressive development in recent years, RNA nanotechnology is still quite limited and its programmability and complexity could not rival the degree of its closely related cousin: DNA nanotechnology. Novel strategies are needed for programmed RNA self-assembly. Here, we have assembled RNA nanocages by re-engineering a natural, biological RNA motif: the packaging RNA of phi29 bacteriophage. The resulting RNA nanostructures have been thoroughly characterized by gel electrophoresis, cryogenic electron microscopy imaging and dynamic light scattering. RNA has a unique position among biomacromolecules. It is relatively simple compared with protein, but more complex than DNA in terms of both structural diversity and functionality. Canonical RNA interactions can be reliably predicted on the basis of simple base-pairing rule (A/G-U & G-C) and well-defined A-conformation RNA duplex. Such simplicity could facilitate the design and construction of RNA nanostructures. RNA also possesses a wide array of tertiary structures and functionalities [1] , [2] , pointing to the possibility of designing complex RNA nanostructures with a wide range of biochemical properties. In the last decade, great efforts have been devoted into this direction and various rationally designed RNA nanostructures have been reported [3] , [4] , [5] , [6] , [7] , [8] , [9] , [10] , [11] , [12] , [13] . RNA nanostructures have further been explored for biomedical applications, for example, small interfering RNA delivery [14] , [15] , [16] and organization of chemical reactions in cells [17] . However, the scope and complexity of accessible RNA nanostructures are quite limited compared with their closely related DNA nanostructures [18] , [19] , [20] , [21] , [22] and novel strategies are needed. Herein we report the assembly of RNA nanocages by re-engineering a natural RNA molecule: the packaging RNA (pRNA) of phi29 bacteriophage. The overall strategy is similar to a previously reported strategy [6] , but showing that this can be extended to other RNA building motifs. pRNA plays an essential role in genomic DNA packaging for phi29 bacteriophage [23] , [24] , [25] . It has received extensive biochemical and structural studies [23] , [24] , [25] , [26] , [27] , [28] . 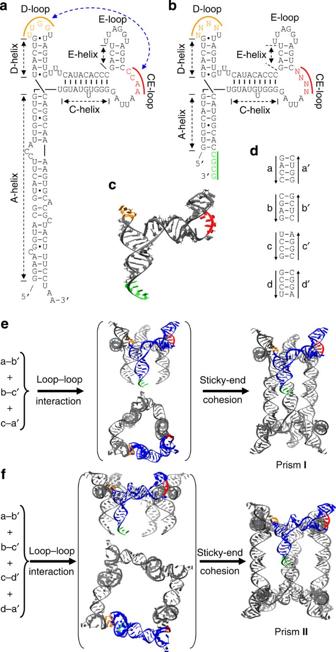Figure 1: Self-assembly of RNA nanoprisms I and II by re-engineering pRNA. (a) Secondary structure of the wild-type pRNA (packaging RNA of bacteriophage phi29). CE- and D-loops can interact with each other via the highlighted, complementary bases (red and golden). (b) Re-engineered pRNA molecules: shortened A-helix with a self-complementary sticky-end (green) and mutated CE- and D-loops (red and golden). (c) A 3D model of pRNA mutants. (d) Four pairs of complementary sequences used for the interacting loops of the pRNA mutants. Self-assembly of (e) a triangular RNA prism (I) and (f) a tetragonal prism (II). pRNAs can bind to each other through both loop–loop interaction and sticky-end cohesion. The mutant pRNAs are named according to the interacting loop sequence; for example, pRNA a–b′ has sequences a at CE-loop (red bases) and b′ at D-loop (golden bases). Figure 1a shows the secondary structure of pRNA. It consists of helical domains and single-stranded internal loops, which are organized into three branches. CE- and D-loops can interact with each other predicted by canonical base pairing. Such loop–loop interaction allows multiple copies of pRNA molecules to associate with each other to form a ring structure. The loop sequence can be mutated. As long as sequence complementarity is satisfied, the loop–loop interaction will be preserved. While the ring size (pentamer [28] versus hexamer [24] , [25] ) is still in debate for the biological phi29 packaging motor, pRNA will self-associate into different-sized oligomers in vitro . This phenomenon highlights the structural flexibility of pRNA. In addition to its native biological role, pRNA has been successfully used as an effective carrier for small RNA delivery [29] , [30] , [31] . Due to such biomedical applications, pRNA has been explored as a building block for nanoconstruction [12] , [13] . As a building block, pRNA is a versatile RNA motif. It has many independent variables (lengths of duplex domains A, C, D and E; interaction loop sequences; and the three-way junction angles), which could potentially allow it to construct sophisticated nanostructures. However, no structurally well-defined pRNA nanostructures beyond small circular oligomers have been constructed so far. Herein, we demonstrate that pRNA can be re-engineered to self-assemble into a series of structurally well-defined nanocages, specifically nanoprisms. The resulting RNA nanostructures have been thoroughly characterized by gel electrophoresis, cryogenic electron microscopy (cryoEM) and dynamic light scattering (DLS). Figure 1: Self-assembly of RNA nanoprisms I and II by re-engineering pRNA. ( a ) Secondary structure of the wild-type pRNA (packaging RNA of bacteriophage phi29). CE- and D-loops can interact with each other via the highlighted, complementary bases (red and golden). ( b ) Re-engineered pRNA molecules: shortened A-helix with a self-complementary sticky-end (green) and mutated CE- and D-loops (red and golden). ( c ) A 3D model of pRNA mutants. ( d ) Four pairs of complementary sequences used for the interacting loops of the pRNA mutants. Self-assembly of ( e ) a triangular RNA prism ( I ) and ( f ) a tetragonal prism ( II ). pRNAs can bind to each other through both loop–loop interaction and sticky-end cohesion. The mutant pRNAs are named according to the interacting loop sequence; for example, pRNA a–b′ has sequences a at CE-loop (red bases) and b′ at D-loop (golden bases). Full size image RNA Nanoprisms I and II The current strategy is built on three aspects of pRNA: (1) well-established secondary structure, (2) reliably predictable loop–loop interaction among pRNA molecules and (3) sufficient structural flexibility at the three-way junction. Figure 1 illustrates our design. In the case of triangular prism ( I ) design, we have constructed three mutant pRNAs (a–b′, b–c′, c–a′) whose 3′ ends (at A-helix) have been elongated by four self-complementary bases (green). Except the two interacting CE- and D-loops and the 3′ tail, all mutants have the same sequence as the wild-type pRNA. The mutants are dubbed according to the two interacting loops sequences, for example, pRNA a–b′ has sequences a for CE-loop (red) and b′ for D-loop (golden). a/a′, b/b′, and c/c′ are three pairs of complementary sequences ( Fig. 1d ). When co-existing, the three RNA molecules will recognize and bind to each other through sequence-specific loop–loop interactions to form a trimeric ring structure. The 3′ tail (GCGC, green) has a palindromic sequence. Hybridization between two such tails leads two RNA molecules to associate with each other at the A-helix domains. The length (20 basepairs) of the resulted, fused A-helix (including the sticky-end region) is carefully chosen in such a way that any A-helix cohesion brings two trimeric rings to face each other and allows the other two pairs of A-helix ends to hybridize with each other. The dimerization of two trimeric rings forms a triangular prism (Prism I; containing six RNA molecules) with the two trimeric rings as its top and bottom faces. Similarly, a tetragonal prism (Prism II ; containing eight RNA molecules) can be assembled from four types of RNA molecules (a–b′, b–c′, c–d′, and d–a′). RNA assembly is carried out by a simple cooling process in a neutral, Mg 2+ -containing aqueous buffer. Equal ratio of RNA molecules are mixed and cooled from 60 °C to 4 °C over 3.5 h. After assembly, the RNA complexes are either analysed by native polyacrylamide gel electrophoresis (native PAGE) directly or visualized by cryoEM upon concentrating. Native PAGE has been proven as an effective technique for characterization of DNA/RNA nanostructures. To determine the chemical identities of the assembled RNA complexes in PAGE, we have prepared a series of reference samples, particularly, blunt-ended RNA molecules (a–b′+b–c′+c–a′) b and (a–a′) b that lack 3′ sticky ends. They can oligomerize into circular rings via loop–loop interaction but the circular rings cannot further dimerize into nanoprisms. For each design, at the correct composition, one dominant sharp band appears and has the expected electrophoretic mobility when compared with all reference complexes, suggesting that the major band is the designed RNA nanoprism ( Fig. 2 ). Please note that when pRNAs are partially complementary to each other (for example, a–b′+b–c′ or b–c′+c–a′ or c–a′+a–b′), they may form intermediate complexes. Their stabilities depend on the exact loop sequences which determine the strength of the loop–loop interactions. Stable complexes (b–c′+c–a′ and c–a′+a–b′) appear as sharp bands and an unstable complex (a–b′+b–c′) smears out. We have estimated the assembly yields for both prisms with Image J [32] , an image-processing software, from the band intensities. The yields are 89.5% and 81.1% for prisms I and II , respectively. We noticed that though the desired nanoprisms were stable and shown as sharp bands, the individual RNA molecules and some partial complexes (for references) could weakly associate with each other and appeared as smear or multiple weak bands. 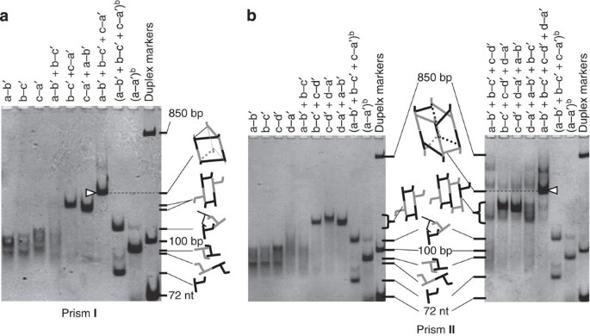Figure 2: Native polyacrylamide gel electrophoresis (PAGE) of RNA prisms I (a) and II (b). Sample compositions are indicated above the gel images and the chemical identity of each band is suggested at the sides of the gels. Arrowheads indicate the targeted prisms. Note that (a–b′+b–c′+c–a′)band (a–a′)bare made from RNA molecules without sticky ends. In the lane of (a–b′+b–c′+c–a′)b, extra amount of (a–b′)bis added to show the mobility of individual pRNA. Figure 2: Native polyacrylamide gel electrophoresis (PAGE) of RNA prisms I (a) and II (b). Sample compositions are indicated above the gel images and the chemical identity of each band is suggested at the sides of the gels. Arrowheads indicate the targeted prisms. Note that (a–b′+b–c′+c–a′) b and (a–a′) b are made from RNA molecules without sticky ends. In the lane of (a–b′+b–c′+c–a′) b , extra amount of (a–b′) b is added to show the mobility of individual pRNA. Full size image To reveal the 3D (three-dimensional) structures of the assembled RNA complexes, we have visualized the RNA complexes by cryoEM ( Figs 3 and 4 ). This powerful, biophysical technique can reveal the structural details of biomacromolecules in their native conformations. In the raw images, individual RNA complexes can be easily identified (indicated by white boxes). Their shapes resemble the expected two-dimensional projections of the designed prism structures. With the observed individual RNA particles, we have applied a single particle 3D reconstruction technique [33] , [34] to reconstruct the original 3D structures of the RNA complexes. This process resulted in structural models of prisms I and II at resolutions of 3.2 and 1.6 nm, respectively. To verify those structural models, two comparisons have been performed: the computed two-dimensional projections with individual particles ( Figs 3c and 4c ) and with class average of raw particles with similar views ( Supplementary Figs 1 and 2 ). Clear similarities could be seen in those comparisons. Furthermore, the measured prism dimensions have good agreement with the designs ( Supplementary Fig. 3 ). Thus, the reconstructed structures truly represent the native conformation of the RNA complexes. 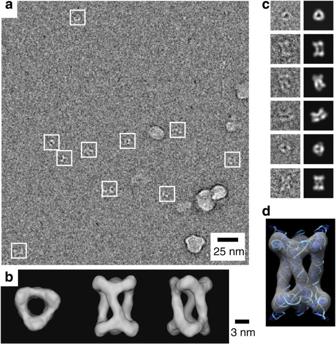Figure 3: CryoEM analysis of triangular RNA prism I. (a) A raw cryoEM (cryogenic electron microscopy) image. White boxes indicate individual RNA complexes. (b) Three views of the triangular prism model reconstructed from cryoEM images. (c) Comparison between individual raw particles and computer-generated two-dimensional projections of the 3D model in similar orientations. (d) Fitting of the pRNA crystal structure27into the cryoEM density map of prismI. Figure 3: CryoEM analysis of triangular RNA prism I. ( a ) A raw cryoEM (cryogenic electron microscopy) image. White boxes indicate individual RNA complexes. ( b ) Three views of the triangular prism model reconstructed from cryoEM images. ( c ) Comparison between individual raw particles and computer-generated two-dimensional projections of the 3D model in similar orientations. ( d ) Fitting of the pRNA crystal structure [27] into the cryoEM density map of prism I . 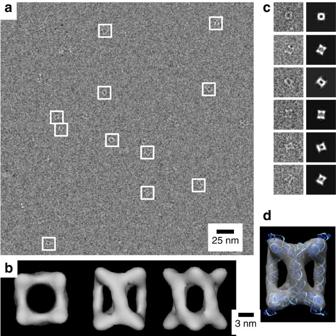Figure 4: CryoEM analysis of tetragonal RNA prism II. (a) A raw cryoEM image. White boxes indicate individual RNA complexes. (b) Three views of the tetragonal prism model reconstructed from cryoEM images. (c) Comparison between individual raw particles and computer-generated two-dimensional projections of the 3D model in similar orientations. (d) Fitting of pRNA crystal structure into the cryoEM density map of prismII. Full size image Figure 4: CryoEM analysis of tetragonal RNA prism II. ( a ) A raw cryoEM image. White boxes indicate individual RNA complexes. ( b ) Three views of the tetragonal prism model reconstructed from cryoEM images. ( c ) Comparison between individual raw particles and computer-generated two-dimensional projections of the 3D model in similar orientations. ( d ) Fitting of pRNA crystal structure into the cryoEM density map of prism II . Full size image RNA Nanoprism III pRNA is a versatile structural platform and can be modified in different ways to construct different nanostructures. For example, we reason that if sticky end is added to E-helix instead of A-helix, the oligomeric rings can dimerize to form prism as well ( Fig. 5 ). To test this hypothesis, we re-engineered the pRNA as following: (i) capping the A-helix with a UUUU loop (A-loop), (ii) removing E-loop from E-helix and (iii) adding a sticky end (GCGC, green) to the 3′ end of E-helix. Such modifications will not interfere with the interaction between D- and CE-loops because both A- and E-helixes are distant from the loop–loop interaction. The mutant pRNA molecules can still bind to each other via loop–loop interaction to form circular oligomers, which would further dimerize through E-helix sticky-end cohesion to form prisms. If this reasoning is correct, three such mutant RNA molecules *a–b′, *b–c′ and *c–a′ will self-assemble into a triangular prism ( III ). 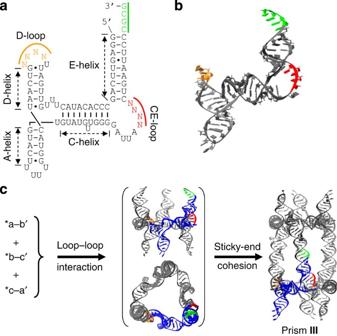Figure 5: Self-assembly of RNA nanoprism III by re-engineering pRNA. (a) A re-engineered pRNA molecule: capping A-helix with a loop and adding a self-complementary sticky end (green) to E-helix. (b) Predicted 3D structure of pRNA mutant. (c) Self-assembly of triangular RNA prismIII. * in the name of a pRNA mutant indicates that the RNA has a sticky end on E-helix. Figure 5: Self-assembly of RNA nanoprism III by re-engineering pRNA. ( a ) A re-engineered pRNA molecule: capping A-helix with a loop and adding a self-complementary sticky end (green) to E-helix. ( b ) Predicted 3D structure of pRNA mutant. ( c ) Self-assembly of triangular RNA prism III . * in the name of a pRNA mutant indicates that the RNA has a sticky end on E-helix. Full size image Prism III efficiently assembles as designed. Native PAGE shows a dominant, sharp band with the mobility expected for the designed prism III ( Fig. 6 ). From the RNA band intensities, the assembly yield is estimated to be 92.3%. The 3D structure of prism III has been further confirmed by cryoEM imaging, which leads to a 3D structural model at a resolution of 2.8 nm ( Fig. 7 and Supplementary Fig. 4 ). 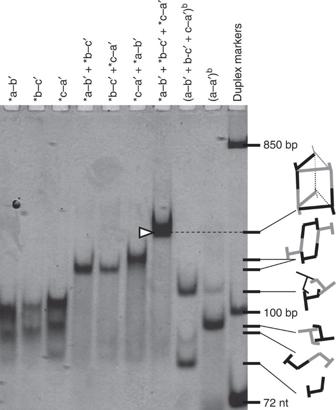Figure 6: Native PAGE of RNA prism III. Sample compositions are indicated above the gel image and the chemical identity of each band is suggested at the sides of the gels. Arrowheads indicate the targeted prisms. Note that (a–b′+b–c′+c–a′)band (a–a′)bare made from RNA molecules without sticky ends. Figure 6: Native PAGE of RNA prism III. Sample compositions are indicated above the gel image and the chemical identity of each band is suggested at the sides of the gels. Arrowheads indicate the targeted prisms. Note that (a–b′+b–c′+c–a′) b and (a–a′) b are made from RNA molecules without sticky ends. 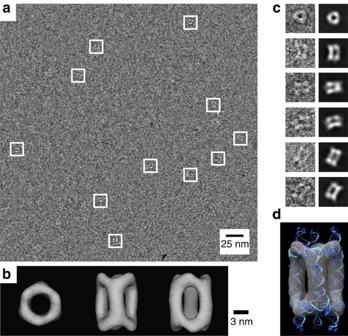Figure 7: CryoEM analysis of triangular RNA prism III. (a) White boxes indicate individual RNA complexes. (b) Three views of the triangular prism model reconstructed from cryoEM images. (c) Comparison between individual raw particles and computer-generated two-dimensional projections of the 3D model in similar orientations. (d) Fitting of pRNA crystal structure into the cryoEM density map of prismIII. Full size image Figure 7: CryoEM analysis of triangular RNA prism III. ( a ) White boxes indicate individual RNA complexes. ( b ) Three views of the triangular prism model reconstructed from cryoEM images. ( c ) Comparison between individual raw particles and computer-generated two-dimensional projections of the 3D model in similar orientations. ( d ) Fitting of pRNA crystal structure into the cryoEM density map of prism III . Full size image Fitting pRNA crystal structure into the nanoprisms High-resolution pRNA crystal structure [27] can fit into the reconstructed prism models ( Figs 3d , 4d and 7d ). In the crystal structure, the pRNA was modified to facilitate its crystallization, including deletion of (i) three bases (AUU) at the 5′ end of the CE-loop and (ii) one base (U) at the 5′ end of D-loop. Thus, the detailed crystal structure of pRNA might be slightly different from the solution structure in our nanoprisms, but the global folding is expected to be the same. Most of the RNA molecules can be easily placed into the cryoEM maps. However, the out-pointing hairpins (E-helix in prism I / II and A-helix in prism III ) cannot be located into the cryoEM map. Those hairpins protruding outside the RNA prisms are not restricted by other segments. Thus, they would have significant degree of conformational freedom and are structurally flexible. Consequently, their electron densities would not be observed by cryoEM. Stability of RNA nanoprisms We have further examined the thermal stability of the assembled RNA prisms by DLS ( Fig. 8 ). Intact prisms exhibit large hydrodynamic diameters at low temperature. As temperature increases, the prisms dissociate into pRNA monomers, leading to the decrease of hydrodynamic diameters. The apparent melting temperatures fall in the range of 37–47 °C. Melting temperature increases in the order of I < II < III . In prisms I and II , pRNA motifs are in similar conformation so it is not a surprise that prisms I and II have similar thermal stability. pRNA motifs in prism III interact with each other quite differently from the other two prisms. Prism III is significantly more thermally stable indicating that the pRNA motif is less strained in this prism. We have also tested their stability against fetal bovine serum ( Fig. 9 and Supplementary Fig. 5 ). All prisms degrade quite fast. Under current experimental condition, one hour incubation leads to~40%, 80% and 40% degradation for prisms I , II and III , respectively. Prisms I and III degrade much slower than prism II presumably because they are more compact; thus, RNase has less access to RNAs. To improve the chemical stability of the RNA complexes for practical applications, some chemical modifications are needed [16] , [31] . 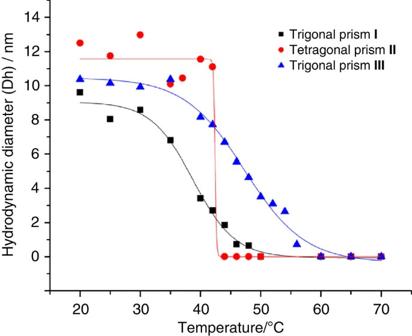Figure 8: Thermal stability study of RNA prisms by dynamic light scattering (DLS). There was a large size change (hydrodynamic diameter, Dh) accompanying the dissociation process from an RNA prism to individual pRNA motifs. Figure 8: Thermal stability study of RNA prisms by dynamic light scattering (DLS). There was a large size change (hydrodynamic diameter, Dh) accompanying the dissociation process from an RNA prism to individual pRNA motifs. 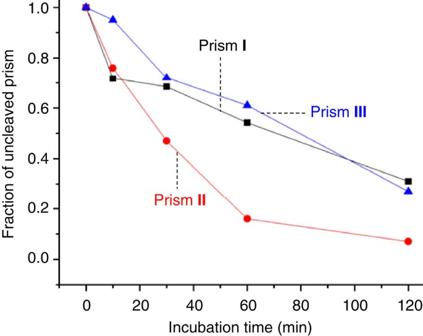Figure 9: Chemical stability of pRNA prisms in fetal bovine serum. Quantified degradation profiles from the PAGE images (Supplementary Fig. 5). Full size image Figure 9: Chemical stability of pRNA prisms in fetal bovine serum. Quantified degradation profiles from the PAGE images ( Supplementary Fig. 5 ). Full size image It would be straight forward to apply this strategy to assemble other polygonal prisms, for example, pentagonal and hexagonal prisms. In the current strategy, a polygonal prism is formed by dimerizing the corresponding polygons. As long as a specific polygon can be constructed, the corresponding polygonal prism can be formed. It has been demonstrated that pRNA pentagon and hexagon could be assembled [24] , thus pentagonal and hexagonal prisms should be readily assembled by the current strategy. In conclusion, we have developed an approach for RNA self-assembly. By re-engineering a native biological RNA molecule, a series of RNA 3D nanocages can be designed and assembled. We expect that this capability would facilitate a wide range of applications of RNA nanotechnology, including as carriers for small RNA delivery [14] , [15] , [16] , [29] , [30] , [31] , and as scaffold hubs for in vivo organization of biomacromolecules [17] and nanoparticles [35] . We are currently investigating whether the natural interacting RNA motifs can be further explored to design novel RNA motif to provide a new platform for RNA nanoconstruction. Oligonucleotides All DNA strands were purchased from IDT, Inc. and purified by 10% denaturing PAGE. RNA sequences were adapted from the wild-type phi29 pRNA and were listed below (the interacting loop sequences and the sticky ends were highlighted in the format italics, bold italics and underlines (orange, red and green colour, respectively, as in Figs 1 and 5 ): a–b′: 5′-GUGUCAUGUGUAUGUUGGGGAUUA GACC CUGAUUGAGUUC AGCCCACAUACUUUGUUGAUU CUCG GUCAAUCAUGGCAC CGCG -3′; b–c′: 5′-GUGUCAUGUGUAUGUUGGGGAUUA CGAG CUGAUUGAGUUC AGCCCACAUACUUUGUUGAUU CGGA GUCAAUCAUGGCAC CGCG -3′; c–a′: 5′-GUGUCAUGUGUAUGUUGGGGAUUA UCCG CUGAUUGAGUUC AGCCCACAUACUUUGUUGAUU GGUC GUCAAUCAUGGCAC CGCG -3′; c–d′: 5′-GUGUCAUGUGUAUGUUGGGGAUUA UCCG CUGAUUGAGUUC AGCCCACAUACUUUGUUGAUU AGGC GUCAAUCAUGGCAC CGCG -3′; d–a′; 5′-GUGUCAUGUGUAUGUUGGGGAUUA GCCU CUGAUUGAGUUC AGCCCACAUACUUUGUUGAUU GGUC GUCAAUCAUGGCAC CGCG -3′; *a–b′: 5′-GGAGUUCAGCCCACAUACUUUGUUGAUU CUCG GUCAAUCAU GGUUUUUCAUGUGUAUGUUGGGGAUUA GACC CUGAAUUCC CGCG -3′; *b–c′: 5′-GGAGUUCAGCCCACAUACUUUGUUGAUU CGGA GUCAAUCAU GGUUUUUCAUGUGUAUGUUGGGGAUUA CGAG CUGAAUUCC CGCG -3′; *c–a′: 5′-GGAGUUCAGCCCACAUACUUUGUUGAUU GGUC GUCAAUCAU GGUUUUUCAUGUGUAUGUUGGGGAUUA UCCG CUGAAUUCC CGCG -3′. DNA templates (T7 promoter region is highlighted in bold, the interacting loop sequences and the sticky ends were highlighted in the format bold, italics, bold italics and underlines (blue, orange, red and green colour, respectively, as in Figs 1 and 5 ): For a–b′: 5′- TTCTAATACGACTCACTATA GTGTCATGTGTATGTTGGGG ATTA GACC CTGATTGAGTTCAGCCCACATACTTTGTTGATT CTCG GTC AATCATGGCAC CGCG -3′/5′- CGCG GTGCCATGATTGAC CGAG AATCAA CAAAGTATGTGGGCTGAACTCAATCAG GGTC TAATCCCCAACATACA CATGACAC TATAGTGAGTCGTATTAGAA -3′; For b–c′: 5′- TTCTAATACGACTCACTATA GTGTCATGTGTATGTTGGGG ATTA CGAG CTGATTGAGTTCAGCCCACATACTTTGTTGATT CGGA GTC AATCATGGCAC CGCG -3′/5′- CGCG GTGCCATGATTGAC TCCG AATCAA CAAAGTATGTGGGCTGAACTCAATCAG CTCG TAATCCCCAACATACA CATGACAC TATAGTGAGTCGTATTAGAA -3′; For c–a′: 5′- TTCTAATACGACTCACTATA GTGTCATGTGTATGTTGGGG ATTA TCCG CTGATTGAGTTCAGCCCACATACTTTGTTGATT GGTC GTC AATCATGGCAC CGCG -3′/5′- CGCG GTGCCATGATTGAC GACC AATCAA CAAAGTATGTGGGCTGAACTCAATCAG CGGA TAATCCCCAACATACA CATGACAC TATAGTGAGTCGTATTAGAA -3′; For c–d′: 5′- TTCTAATACGACTCACTATA GTGTCATGTGTATGTTGGGG ATTA TCCG CTGATTGAGTTCAGCCCACATACTTTGTTGATT AGGC GTC AATCATGGCAC CGCG -3′/5′- CGCG GTGCCATGATTGAC GCCT AATCAA CAAAGTATGTGGGCTGAACTCAATCAG CGGA TAATCCCCAACATACA CATGACAC TATAGTGAGTCGTATTAGAA -3′; For d–a′: 5′- TTCTAATACGACTCACTATA GTGTCATGTGTATGTTGGGG ATTA GCCT CTGATTGAGTTCAGCCCACATACTTTGTTGATT GGTC GTC AATCATGGCAC CGCG -3′/5′- CGCG GTGCCATGATTGAC GACC AATCAA CAAAGTATGTGGGCTGAACTCAATCAG AGGC TAATCCCCAACATACA CATGACAC TATAGTGAGTCGTATTAGAA -3′; For *a–b′: 5′- TTCTAATACGACTCACTATA GGAGTTCAGCCCACATACT TTGTTGATT CTCG GTCAATCATGGTTTTTCATGTGTATGTTGGGGATT A GACC CTGAATTCC CGCG -3′/5′- CGCG GGAATTCAG GGTC TAATCCCC AACATACACATGAAAAACCATGATTGAC CGAG AATCAACAAAGTATG TGGGCTGAACTCC TATAGTGAGTCGTATTAGAA -3′; For *b–c′: 5′- TTCTAATACGACTCACTATA GGAGTTCAGCCCACATACT TTGTTGATT CGGA GTCAATCATGGTTTTTCATGTGTATGTTGGGGATT A CGAG CTGAATTCC CGCG -3′/5′- CGCG GGAATTCAG CTCG TAATCCCC AACATACACATGAAAAACCATGATTGAC TCCG AATCAACAAAGTAT GTGGGCTGAACTCC TATAGTGAGTCGTATTAGAA -3′; For *c–a′: 5′- TTCTAATACGACTCACTATA GGAGTTCAGCCCACATACT TTGTTGATT GGTC GTCAATCATGGTTTTTCATGTGTATGTTGGGGATT A TCCG CTGAATTCC CGCG -3′/5′- CGCG GGAATTCAG CGGA TAATCCCC AACATACACATGAAAAACCATGATTGAC GACC AATCAACAAAGTATG TGGGCTGAACTCC TATAGTGAGTCGTATTAGAA -3′. RNA preparation All RNA molecules were synthesized by in vitro transcription with T7 RNA polymerase (the AmpliScribe T7-Flash transcription kit; Epicenter, Inc.) from corresponding DNA templates by following the manufacturer-recommended protocol, and then purified by the 10% denaturing PAGE. Formation of pRNA prisms For assembly of triangular prisms I and III , all component strands at 500 nM were combined in TAE/Mg 2+ buffer and incubated at 60 °C for 5′, 50 °C for 30′, 37 °C for 30′, 22 °C for 30′ and 4 °C for 2 h. TAE/Mg 2+ buffer contained 40 mM Tris base (pH 8.0), 20 mM acetic acid, 2 mM EDTA and 12.5 mM Magnesium Acetate. For assembly of prism II , we first separately hybridized d–a′+a–b′ and b–c′+c–d′ (500 nM for each strand) by incubation at 60 °C for 5′, 50 °C for 30′, 37 °C for 30′, 22 °C for 30′ and 4 °C for 2 h. Then these two complexes (equal volumes) were combined and incubated at 37 °C for 30′, 22 °C for 30′ and 4 °C for 2 h. Denaturing PAGE A 10% denaturing PAGE gel was prepared with the 19:1 acrylamide/bisacrylamide gel, 8 M urea, and TBE buffer (89 mM Tris base (pH=8.0), 89 mM boric acid, 2 mM EDTA]. The gel was run at 55 °C for 2 h at 650 V on Hoefer SE 600 electrophoresis system and then stained with ethidium bromide (Sigma). The major band was cut under UV light and eluted out. Native PAGE A 5% native PAGE gel is prepared with the 19:1 acrylamide/bisacrylamide gel and TAE/Mg 2+ buffer. The gel was run at 4 °C, stained with Stains-All (Sigma) and scanned by an office HP scanner. Yield estimation Native PAGE images were analysed by computer software, Image J. After background subtraction of native PAGE images, the lanes of a–b′+b–c′+c–a′ and a–b′+b–c′+c–d′+d–a′ ( Fig. 2 ) and *a–b′+*b–c′+*c–a′ ( Fig. 6 ) were selected, plotted and analysed. The intensities of all bands in the lanes were measured and the yields of prisms were estimated according to the intensity percentages of major bands. Thermal stability study by DLS DLS measurements were carried out with 100 μl 100 nM pRNA prism solutions on Malvern Zetasizer Nano-ZS (Malvern Instruments, UK) at light wavelength of 633 nm at designated temperature in the range of 20–70 °C. At each temperature, the sample was incubated for 10 min before the measurement and ten parallel measurements were tested. Stability assay in serum pRNA prism (1 μg in 30 μl TAE/Mg 2+ buffer) was combined with 20 μl DMEM medium (containing 10% fetal bovine serum (Sigma) and supplemented with 12.5 mM MgCl 2 ) at 22 °C. After incubated for designated duration, the samples were analysed by the 5% native PAGE at 4 °C for 2 h. CryoEM imaging The as-formed RNA complexes were first concentrated to 12 μM with Micron-30 (30 kDa) centrifugal filters. Then 3 μl of each samples were deposited on the Quantifoil grid (Electron Microscopy Sciences, Q250-CR2-400). The grid was blotted with two pieces of filter paper (Whatman, 1001-055) and immediately flash frozen by the liquid nitrogen-cooled liquid ethane. Images were taken on FEI CM200 TEM with accelerating voltage of 200 kV under low-dose condition to minimize radiation damages to the samples. To enhance the image contrast, under-focus in the range of 2–4 μm were used to record the images by films. Single-particle reconstruction The single particle reconstruction was carried out using EMAN 2 software [33] . For all three prisms, about 400 randomly selected individual particles were used to generate 12 class averages to build initial models. The initial orientations of individual particles were randomly assigned within the corresponding asymmetric units of the D3 symmetry for prism I and III, and of D4 symmetry for prism II. Then 850, 1,200 and 700 particles were used for the refinements of prisms I, II and III, respectively. The refinements were carried out with a 2-degree angle interval. A projection matching algorithm was applied for the determination of the center and orientation of raw particles in the iterative refinement for each prism. The corresponding symmetries were imposed during the reconstructions. The resolutions of resulted structural density maps were determined to be at 3.2, 1.6 and 2.8 nm for prisms I, II and III, respectively, with the Fourier shell correlation (0.5 threshold criterion) of two 3D maps separately built from even and odd halves of the data sets. Final reconstruction results were visualized by UCSF Chimera software [34] . Modelling and fitting All prism models were built from a crystal structure of pRNA mutant (PDB ID: 3R4F) and idealized A-form RNA duplex with computer software Coot [36] . In the crystal, pRNA mutant formed a tetrameric ring in the crystal. For prism II, tetrameric 3R4F were directly used as the top and bottom faces for the model building and all A-helix domains were elongated to the designed length in Coot. The top and bottom faces were fitted into the prism II electron density map separately with ‘fit in map’ function in Chimera. The model overall fitted the cryoEM map and the lengths of the model prism II edges (20 bp) matched well with the map. The prism II model was further modified to better fit into the map by adding flexibility at the three-way junction point, where A-helix domain and the rest of 3R4F were separately fit into the map by rigid body fit in Coot and then linked together. The geometry and phase of each domain did not have any significant change during the refinement and fitting. At last, the bond lengths and angles of prism II model were idealized in Coot to generate the prism II final model. For prism I, a trimer of 3R4F was first built in Coot by applying 3-fold rotation symmetry on one 3R4F molecule along the rotation axis and then modified at the loop–loop interaction structure in accordance with the counterpart in the crystal. Afterward, two trimers of 3R4F were used to build the prism I model and fit into the cryoEM map following the procedures described for prism II. For prism III, the 3R4F molecule was first modified according to the design to add a UUUU loop at the A-helix as well as to open and elongate the E-helix. A computed UUUU structure [37] was used here for capping A-helix and an idealized A-form RNA was applied for E-helix elongation in Coot. After reconstruction of prism III building motif, a trimer of the motifs was generated similarly as described for prism I. Then two trimers of prism III motifs were built and fit into the cryoEM map by following the method described for prism II. How to cite this article: Hao, C. et al. Construction of RNA nanocages by re-engineering the packaging RNA of Phi29 bacteriophage. Nat. Commun. 5:3890 doi: 10.1038/ncomms4890 (2014).